Molecular basis for erythromycin-dependent ribosome stalling during translation of the ErmBL leader peptide In bacteria, ribosome stalling during translation of ErmBL leader peptide occurs in the presence of the antibiotic erythromycin and leads to induction of expression of the downstream macrolide resistance methyltransferase ErmB. The lack of structures of drug-dependent stalled ribosome complexes (SRCs) has limited our mechanistic understanding of this regulatory process. Here we present a cryo-electron microscopy structure of the erythromycin-dependent ErmBL-SRC. The structure reveals that the antibiotic does not interact directly with ErmBL, but rather redirects the path of the peptide within the tunnel. Furthermore, we identify a key peptide–ribosome interaction that defines an important relay pathway from the ribosomal tunnel to the peptidyltransferase centre (PTC). The PTC of the ErmBL-SRC appears to adopt an uninduced state that prevents accommodation of Lys-tRNA at the A-site, thus providing structural basis for understanding how the drug and the nascent peptide cooperate to inhibit peptide bond formation and induce translation arrest. During protein synthesis, nascent polypeptide chains can modulate the efficiency of translation [1] . Nascent polypeptide-mediated translation regulation can be an intrinsic property of the nascent chain [1] or can depend on the additional presence of a ligand, for example, a macrolide antibiotic such as erythromycin (ERY) [2] , [3] . Biochemical and genetic studies of several drug-dependent regulatory peptides have provided initial models for how interactions within the ribosomal tunnel can relay back to the peptidyltransferase centre (PTC) to induce translation arrest [2] , [3] . Interestingly, biochemical characterization of distinct Erm leader peptide-stalled ribosome complexes (SRCs) indicates that fundamental differences exist in their mechanisms of translational arrest: for example, mutations of 23S rRNA nucleotides A2062 and A2503 abolish stalling with ErmAL1 and ErmCL, but have no influence on ErmBL- and ErmDL-mediated translation arrest [4] . Furthermore, different regulatory peptides appear to have a different sensitivity to the chemical structure of the antibiotic [4] , [5] , [6] . The lack of structural information has made it difficult to explain these conceptually important distinctions and provide models of drug-dependent stalling to a sufficient level of molecular detail. Here we have characterized structurally and biochemically the requirements for ribosome stalling during translation of the ErmBL leader peptide. Similar to other inducible macrolide resistance genes, ermB is controlled by programmed arrest of translation of the leader peptide ErmBL ( Fig. 1a ). Previous studies demonstrated that polymerization of the ErmBL nascent chain halts when the Asp codon (D10) of the ermBL open-reading frame (ORF) enters the ribosomal P-site and the Lys (K11) codon is placed in the A-site [4] , [7] ( Fig. 1a ). Consistently, our findings indicate that the ErmBL-SRC contains an ErmBL-transfer RNA in the P-site and Lys-tRNA in the A-site, and thus stalling results from inability of the ribosome to catalyse peptide bond formation. On the basis of our cryo-electron microscopy (EM) structure of the ErmBL-SRC, we suggest that peptide bond formation does not occur because the accommodation of Lys-tRNA at the A-site of the PTC is corrupted. Moreover, we identify critical residues in ErmBL and in the ribosome, which we propose to be important for maintaining the PTC in an uninduced and thus inactive state. 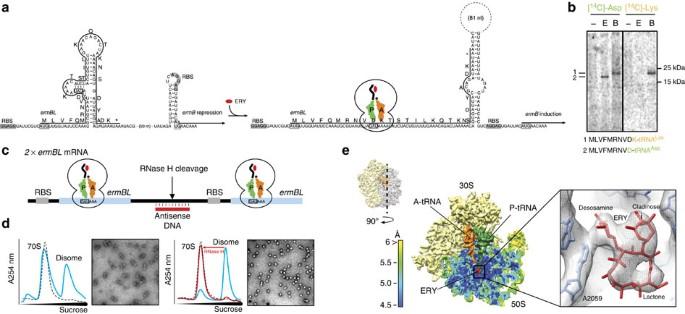Figure 1: Cryo-EM structure of the ErmBL-stalled ribosome complex. (a) Schematic forermBL-dependent regulation ofermBtranslation in the presence of erythromycin (ERY). (b)In vitrotranslation of ErmBL using either14C-Asp or14C-Lys in the absence (−) or presence (E) of 50 μM ERY. In the control samples (B), where translation was carried out in the absence of ERY, but in presence of borrelidin (a Thr-tRNA synthetase inhibitor), translation arrest occurred after an 11-amino-acid nascent chain was polymerized (such that codon 12 is in the A-site, which is one codon further compared with the natural stall site), thereby providing a mobility marker and confirming14C-Lys incorporation in the absence of ERY. (c) The bicistronic 2 ×ermBLmRNA was translatedin vitroin the presence of 10 μM ERY to generate ErmBL-SRC disomes. (d) Complementary DNA oligo and RNase H cleavage converts disomes to monosomes, as shown by sucrose density centrifugation and negative stain EM. (e) Surface and cross-section of the ErmBL-SRC, containing 30S (yellow), 50S (coloured according to local resolution), A-tRNA (orange), P-tRNA (green) and ERY (red). Inset shows electron density for ERY (grey mesh) with fitted crystal structure (PDB3OFR)11. Figure 1: Cryo-EM structure of the ErmBL-stalled ribosome complex. ( a ) Schematic for ermBL -dependent regulation of ermB translation in the presence of erythromycin (ERY). ( b ) In vitro translation of ErmBL using either 14 C-Asp or 14 C-Lys in the absence (−) or presence (E) of 50 μM ERY. In the control samples (B), where translation was carried out in the absence of ERY, but in presence of borrelidin (a Thr-tRNA synthetase inhibitor), translation arrest occurred after an 11-amino-acid nascent chain was polymerized (such that codon 12 is in the A-site, which is one codon further compared with the natural stall site), thereby providing a mobility marker and confirming 14 C-Lys incorporation in the absence of ERY. ( c ) The bicistronic 2 × ermBL mRNA was translated in vitro in the presence of 10 μM ERY to generate ErmBL-SRC disomes. ( d ) Complementary DNA oligo and RNase H cleavage converts disomes to monosomes, as shown by sucrose density centrifugation and negative stain EM. ( e ) Surface and cross-section of the ErmBL-SRC, containing 30S (yellow), 50S (coloured according to local resolution), A-tRNA (orange), P-tRNA (green) and ERY (red). Inset shows electron density for ERY (grey mesh) with fitted crystal structure (PDB3OFR) [11] . Full size image Cryo-EM structure of the ErmBL-SRC To assess whether the ErmBL-SRC contains the nascent chain attached to tRNA Asp in the P-site or to tRNA Lys in the A-site, in vitro translation of ErmBL was performed in the presence of ERY and either radiolabelled aspartate or lysine. Analysis of the ErmBL nascent chain shows that radiolabelled Asp, but not Lys, was incorporated into the peptidyl-tRNA of the SRC ( Fig. 1b ). Thus, the ribosome stalls because it is unable to catalyse formation of a peptide bond between the 10-amino-acid-long ErmBL nascent chain attached to the tRNA Asp in the P-site and the incoming Lys-tRNA Lys ( Fig. 1a ). To unravel the structural basis for ErmBL-mediated stalling, we generated ErmBL-SRC for analysis using cryo-EM. For previous structures of drug-independent SRCs, the nascent chains were of sufficient length to exit the ribosomal tunnel, enabling purification of the SRC using N-terminal affinity tags [8] , [9] , [10] . In contrast, the peptides controlling macrolide resistance genes, including the 10-amino-acid-long ErmBL nascent chain, are too short to exit the tunnel, making preparation of SRC by N-terminal affinity tagging impossible. Consequently, we established a SRC purification technique employing a bicistronic (2 × ermBL ) messenger RNA (mRNA) bearing two ermBL ORFs. The ORFs were separated by a 22-nucleotide linker and each had a strong ribosome-binding site (RBS) ( Fig. 1c ). In vitro translation of 2 × ermBL leads to the formation of disomes (one ribosome per cistron, two ribosomes per mRNA), as evident from sucrose gradient analysis and negative-stain EM ( Fig. 1d ). Importantly, disome formation is strictly dependent on the presence of ERY and does not occur on monocistronic ermBL mRNAs ( Supplementary Fig. 1 ). To avoid orientation bias during cryo-EM analysis, the disomes were converted into monosomes by cleavage of the linker using an antisense DNA oligonucleotide and RNase H ( Fig. 1c,d ). Cryo-EM and single-particle reconstruction of the resulting ErmBL-SRC, coupled with in silico sorting ( Supplementary Fig. 2 ), yielded one major homogeneous subpopulation of ribosomes bearing tRNAs in the A- and P-sites ( Fig. 1e ). Local resolution indicates that most of the ErmBL-SRC map, in particular the core region encompassing the PTC and ribosomal tunnel, reaches a resolution of 4.5 Å ( Fig. 1e and Supplementary Fig. 3 ). Consistent with this resolution, distinct features of the electron density for ERY, such as the lactone ring, desosamine and cladinose sugars, can be unambiguously resolved ( Fig. 1e ). Moreover, rigid-body fitting of the crystal structure of ERY in complex with the Escherichia coli ribosome [11] indicates that the drug is bound to its canonical position [11] , [12] in the ErmBL-SRC ( Fig. 1e ). The path of ErmBL through the ribosomal tunnel Additional density in the ErmBL-SRC, which we assign to the ErmBL nascent chain, is observed within the ribosomal tunnel extending from the CCA-end of the P-tRNA ( Fig. 2a ). Unlike the nascent chains of TnaC [8] and SecM [10] that extend throughout the entire length of ribosomal tunnel ( Fig. 2b,c ), the 10-amino-acid-long ErmBL occupies only the upper third of this conduit ( Fig. 2a ). Moreover, the unique path of the ErmBL nascent chain enables it to bypass the tunnel-bound ERY ( Fig. 2d ). In contrast, the nascent chains of SecM- and TnaC-SRC, as well as of other ribosome-nascent chain complexes [9] , [13] , [14] , [15] , adopt conformations that would be sterically obstructed by the drug ( Fig. 2e,f ). Although ermBL translation by the ERY-bound ribosome stalls at the 10th codon, the conformation of the ErmBL polypeptide within the tunnel ( Fig. 2a ) illustrates the general principle of how a specific subset of polypeptides can bypass ERY to be translated on drug-bound ribosomes [16] . 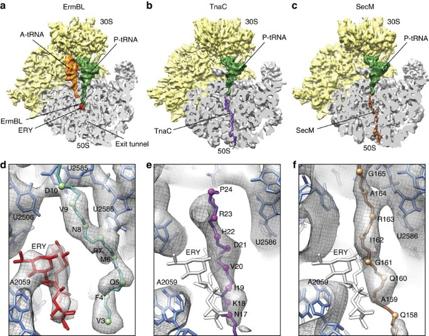Figure 2: Path of the ErmBL compared with TnaC and SecM nascent chains. (a–c) Comparison of cryo-EM structures of ErmBL-SRC, TnaC-SRC8and SecM-SRC10, with a transverse section of the 50S subunit (grey) displaying the path of the respective nascent chains through the ribosomal tunnel. (d–f) Paths of the (d) ErmBL (teal), (e) TnaC8(purple) and (f) SecM10(brown) nascent chains. Erythromycin (ERY)11is coloured red in (d) ErmBL-SRC, whereas the superimposed position of ERY is coloured white in (e) TnaC-SRC and (f) SecM-SRC. Figure 2: Path of the ErmBL compared with TnaC and SecM nascent chains. ( a – c ) Comparison of cryo-EM structures of ErmBL-SRC, TnaC-SRC [8] and SecM-SRC [10] , with a transverse section of the 50S subunit (grey) displaying the path of the respective nascent chains through the ribosomal tunnel. ( d – f ) Paths of the ( d ) ErmBL (teal), ( e ) TnaC [8] (purple) and ( f ) SecM [10] (brown) nascent chains. Erythromycin (ERY) [11] is coloured red in ( d ) ErmBL-SRC, whereas the superimposed position of ERY is coloured white in ( e ) TnaC-SRC and ( f ) SecM-SRC. Full size image Closer examination of the ErmBL-SRC structure indicates an apparent lack of contact between ErmBL and ERY ( Fig. 2d ). This is distinct from the direct interaction between the nascent chain and the drug that was proposed for ErmCL, based on the observation that removal or modification of the C3 cladinose sugar abolishes ErmCL stalling [17] , [18] . Therefore, we tested whether ErmBL stalling is sensitive to structural modifications of the antibiotic cofactor. In excellent agreement with the structural predictions, ErmBL stalling could be induced not only by ERY, but also by a wide range of tunnel-binding macrolides, including those which failed to induce ErmCL-SRC formation [17] , for example, solithromycin, which lacks the C3 cladinose, as well as oleandomycin and ITR-054, which contain alterations of the C3 sugar ( Fig. 3 ). As expected, antibiotics josamycin and clindamycin, which overlap with the A-site and inhibit formation of the first peptide bond [11] , [12] , [19] ( Fig. 3 ), and quinupristin, which overlaps with the path of ErmBL [12] , [20] ( Fig. 3 ), did not allow the drug-bound ribosome to reach the ermBL stall site ( Fig. 3 ). 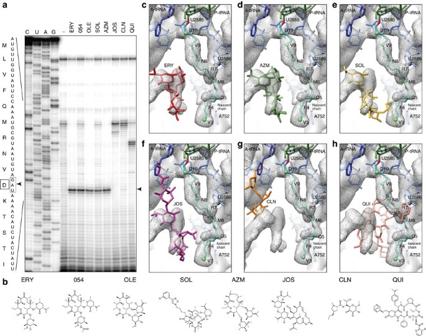Figure 3: Superimposition of various antibiotics relative to ErmBL. (a) Detection of ribosome stalling by toe-printing during translation ofermBL, in the presence of the antibiotics erythromycin (ERY), ITR-054 (054), oleandomycin (OLE), solithromycin (SOL), azithromycin (AZM), josamycin (JOS), clindamycin (CLN) and quinupristin (QUI). The arrowed toe-print band indicates that ErmBL arrests translation with the Asp (D10) codon (boxed) located in the P-site. (b) Chemical structures of ERY, macrolides ITR-054 (054), OLE, the ketolide SOL and the azalide AZM compared with the macrolide JOS, the lincosamide CLN and the streptogramin B QUI. Differences between ERY and respective drugs are highlighted. (c) ErmBL-SRC map (grey mesh) with molecular model for ErmBL-tRNA (teal), 23S rRNA (blue) and ERY (red, PDB3OFR11). (d–h) as in (c), but with relative binding positions of (d) AZM (green, PDB1M1K19), (e) SOL (yellow, PDB3ORB42), (f) JOS (purple, PDB2O44), (g) CLN (orange, PDB3OFZ11) and (h) QUI (pink, PDB1SM1 (ref. 20)20). Figure 3: Superimposition of various antibiotics relative to ErmBL. ( a ) Detection of ribosome stalling by toe-printing during translation of ermBL , in the presence of the antibiotics erythromycin (ERY), ITR-054 (054), oleandomycin (OLE), solithromycin (SOL), azithromycin (AZM), josamycin (JOS), clindamycin (CLN) and quinupristin (QUI). The arrowed toe-print band indicates that ErmBL arrests translation with the Asp (D10) codon (boxed) located in the P-site. ( b ) Chemical structures of ERY, macrolides ITR-054 (054), OLE, the ketolide SOL and the azalide AZM compared with the macrolide JOS, the lincosamide CLN and the streptogramin B QUI. Differences between ERY and respective drugs are highlighted. ( c ) ErmBL-SRC map (grey mesh) with molecular model for ErmBL-tRNA (teal), 23S rRNA (blue) and ERY (red, PDB3OFR [11] ). ( d – h ) as in ( c ), but with relative binding positions of ( d ) AZM (green, PDB1M1K [19] ), ( e ) SOL (yellow, PDB3ORB [42] ), ( f ) JOS (purple, PDB2O44), ( g ) CLN (orange, PDB3OFZ [11] ) and ( h ) QUI (pink, PDB1SM1 (ref. 20) [20] ). Full size image Interaction between ErmBL and the ribosomal tunnel To ascertain which residues of ErmBL interact with the ribosomal tunnel, a model for nascent chain was built ( Fig. 4a ). Since the resolution does not allow us to model sidechains, we present only a backbone model for the ErmBL nascent chain. On the basis of this model, three interactions with the ribosomal tunnel are predicted: one from the C terminus (V9-D10) of ErmBL with U2585, a second in the vicinity of R7 with U2586 and a third between F4 and U2609 ( Fig. 4a ). Local resolution indicates that the C terminus of ErmBL (M6-D10) is very stable, providing more confidence in the placement of the backbone model, whereas in contrast, the N-terminal residues (M1-Q5) are flexible to such an extent that modelling of M1 and L2 was not possible due to lack of density and alternative models for the N-terminal are therefore possible ( Fig. 4b ). Consistently, alanine-scanning mutagenesis of ErmBL demonstrated that C-terminal residues, namely, R7 and V9-D10, are critical for stalling, whereas the N-terminal residues are not ( Fig. 4c ). The most distal contact from the PTC between F4 and U2609 ( Fig. 4a,b ) does not appear to be functionally important because neither the F4A mutation, nor the U2609C alteration affected the efficiency of stalling ( Fig. 4c ; Supplementary Fig. 4 ). 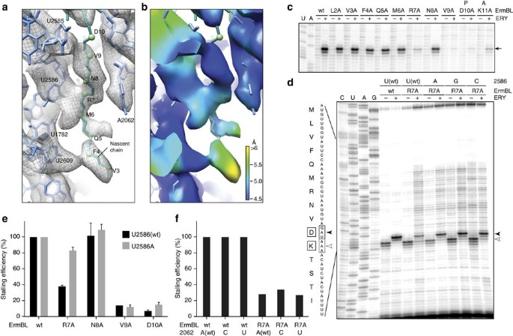Figure 4: Interactions of the ErmBL nascent chain with the ribosome. (a) Interactions of ErmBL (teal) with 23S rRNA (blue) within the exit tunnel of the ribosome. (b) Local resolution map of view shown in (a). (c) Alanine-scanning mutagenesis of ErmBL and effect of mutant peptides on ribosome stalling (arrowed) in the presence (+) and absence (−) of erythromycin (ERY) as determined by toe-printing. (d) Toe-printing of wild type (wt) and mutant (R7A) ErmBL onE. coliribosomes with wt or mutated 23S rRNA nucleotide 2586, in the presence (+) or absence (−) of ERY. All the reactions contained borrelidin, a Thr-tRNA synthetase inhibitor, which, in the absence of ERY-dependent arrest at the Asp (D10) codon, causes translation arrest at the Lys (K11) codon. (e) Influence of the U2586A mutation on stalling efficiency with the wt and mutant ErmBL peptides (an average of two independent experiments; error bars represent the standard deviation of the mean). (f) The mutations of A2062 do not affect ErmBL stalling, nor rescue stalling impaired by the R7A mutation. Figure 4: Interactions of the ErmBL nascent chain with the ribosome. ( a ) Interactions of ErmBL (teal) with 23S rRNA (blue) within the exit tunnel of the ribosome. ( b ) Local resolution map of view shown in ( a ). ( c ) Alanine-scanning mutagenesis of ErmBL and effect of mutant peptides on ribosome stalling (arrowed) in the presence (+) and absence (−) of erythromycin (ERY) as determined by toe-printing. ( d ) Toe-printing of wild type (wt) and mutant (R7A) ErmBL on E. coli ribosomes with wt or mutated 23S rRNA nucleotide 2586, in the presence (+) or absence (−) of ERY. All the reactions contained borrelidin, a Thr-tRNA synthetase inhibitor, which, in the absence of ERY-dependent arrest at the Asp (D10) codon, causes translation arrest at the Lys (K11) codon. ( e ) Influence of the U2586A mutation on stalling efficiency with the wt and mutant ErmBL peptides (an average of two independent experiments; error bars represent the standard deviation of the mean). ( f ) The mutations of A2062 do not affect ErmBL stalling, nor rescue stalling impaired by the R7A mutation. Full size image In contrast, the second contact, between R7 and U2586, plays an important role, since disruption of this interaction by the R7A mutation in ErmBL significantly diminishes stalling ( Fig. 4a,c ). Strikingly, changes in the ribosomal interacting partner (U2586A/G/C) were able to restore the efficiency of translation arrest for the ErmBL-R7A mutant ( Fig. 4d ). The fact that the U2586 mutations (U2586A/G/C) were unable to restore stalling for the ErmBL-V9A or -D10A mutants ( Fig. 4e ) and that stalling of the ErmBL-R7A mutant could not be compensated by alterations of the neighbouring tunnel nucleotide A2062 ( Fig. 4f ) re-emphasizes the specificity and importance of the R7-U2586 interaction for the mechanism of ErmBL stalling. This also provides support for our model for the C-terminal portion of the ErmBL nascent chain and in particular the placement of R7. Notably, the identity of the tunnel nucleotide A2062, which is critical for ErmCL- and ErmAL1-mediated ribosome stalling, was not important for the formation of the ErmBL-SRC [4] , [18] ( Fig. 4e and Supplementary Fig. 4 ). The ErmBL-SRC structure shows the lack of direct contact between A2062 and the nascent chain ( Fig. 4b ), providing a plausible explanation for the clear distinction between the drug-dependent translation arrest directed by different stalling peptides. The conformation of the PTC of the ErmBL-SRC The third contact between the ErmBL nascent chain and the ribosome engages the peptide residues V9/D10 with U2585 of the 23S rRNA. Previous crystallographic analysis of model complexes showed that accommodation of the CCA-end of the A-site tRNA requires movement of the PTC nucleotides U2584 and U2585 to achieve the ‘induced fit’ state of the PTC and provide room for the A-tRNA [21] , [22] , [23] ( Fig. 5a ). The crystal structures of the 50S structure with the PTC in either the uninduced or the induced state were fitted to the electron density for the 50S subunit of the ErmBL-SRC as a rigid body ( Fig. 5a ). Together with difference electron density maps ( Supplementary Fig. 5 ), this procedure suggests that U2584 and U2585 have not shifted sufficiently and remain in an uninduced-like conformation in the ErmBL-SRC, probably due to the interaction of U2585 with the ErmBL nascent chain. The local resolution of the ErmBL map is 4.5 Å, which is sufficient to distinguish movements of 0.9–1.1 Å [24] , [25] , [26] . Because the differences in the nucleotide positions between the induced and uninduced states are in the order of 1–2 Å, we are rather confident that our data would allow us to conclude that the functional state of the PTC in ErmBL-SRC differs from its classic induced state. 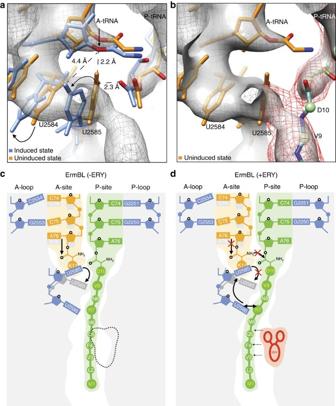Figure 5: The uninduced state of the PTC and an unaccommodated A-tRNA in the ErmBL-SRC prevent peptide bond formation. (a,b) During accommodation of the A-tRNA, U2585 and U2584 undergo conformational changes (arrowed) necessary for peptide bond formation21,22,23. In the ErmBL-SRC, the electron density suggests that U2585 retains an unaccommodated state (orange, PDB1VQ6)21,22,23, thus preventing proper placement of the A-tRNA in the PTC (blue, PDB1VQN)21,22,23. (b) Electron density between the ErmBL nascent chain (dark mesh) and U2585 indicates that the C-terminal amino acids of ErmBL directly interact with U2585, likely restricting its movement. (c,d) Model for the translation of ErmBL (c) in the absence of erythromycin (ERY) (canonical translation), and (d) translation arrest in the presence of ERY (stalling). In (d), the drug restricts the conformational space available for the ErmBL nascent chain such that interactions with U2586 and U2585 are established. We propose that this prevents movement of U2585 from the uninduced to induced state, and thus hinders accommodation of the A-tRNA and peptide bond formation. Figure 5: The uninduced state of the PTC and an unaccommodated A-tRNA in the ErmBL-SRC prevent peptide bond formation. ( a , b ) During accommodation of the A-tRNA, U2585 and U2584 undergo conformational changes (arrowed) necessary for peptide bond formation [21] , [22] , [23] . In the ErmBL-SRC, the electron density suggests that U2585 retains an unaccommodated state (orange, PDB1VQ6) [21] , [22] , [23] , thus preventing proper placement of the A-tRNA in the PTC (blue, PDB1VQN) [21] , [22] , [23] . ( b ) Electron density between the ErmBL nascent chain (dark mesh) and U2585 indicates that the C-terminal amino acids of ErmBL directly interact with U2585, likely restricting its movement. ( c , d ) Model for the translation of ErmBL ( c ) in the absence of erythromycin (ERY) (canonical translation), and ( d ) translation arrest in the presence of ERY (stalling). In ( d ), the drug restricts the conformational space available for the ErmBL nascent chain such that interactions with U2586 and U2585 are established. We propose that this prevents movement of U2585 from the uninduced to induced state, and thus hinders accommodation of the A-tRNA and peptide bond formation. Full size image Although higher resolution will be necessary to validate the exact placement of the PTC residues, its deviation from the fully functional state in the ErmBL-SRC and unaccommodated state of the A-tRNA ( Fig. 5a ) provide an explanation for the translational arrest, since the fully accommodated state is required for efficient nucleophilic attack and fast peptide bond formation ( Fig. 5b ). Moreover, an unaccommodated state of A-tRNA in the ErmBL-SRC is consistent with the finding that Lys encoded by the A-site codon of the SRC is not incorporated into the ErmBL nascent chain ( Fig. 1b ). Although the density corresponding to the A-site amino acid was mostly lacking, we verified biochemically that the A-site tRNA fully retains its aminoacyl moiety through the entire purification protocol ( Supplementary Fig. 6 ). Therefore, we believe that the lack of density reflects the flexibility of the Lys residue of the A-tRNA and reinforces the notion of the ‘inappropriate’ placement of the PTC acceptor substrate ( Fig. 5a,b ). Because the ribosome accelerates peptide bond formation primarily through accurate positioning of the reacting components [27] , [28] , high flexibility of the acceptor substrate would be incompatible with fast peptidyl transfer. Mutation of the SRC acceptor amino acid from lysine to alanine reduced the efficiency of translation arrest ( Fig. 4c ), suggesting that the nature of the A-tRNA amino acid influences the ability of aminoacyl-tRNA to be accommodated in the A-site. Our biochemical and structural insights allow us to propose a model for the concerted action of the drug and the nascent chain in inhibiting the PTC functions: During canonical translation, for example, of ErmBL in the absence of ERY, the nascent polypeptide chain passes freely through the ribosomal tunnel, exploring many conformations most of which are compatible with efficient peptide bond formation. However, in the presence of the macrolide molecule, the path of the nascent chain is restricted because some of the previously accessible routes are obstructed by the drug. In the constrained conformational space the peptide is compelled to establish specific and long-lived contacts with the tunnel wall (R7-U2586) and at the PTC (V9-D10 with U2585) ( Fig. 5c ). These contacts stabilize the improper (uninduced) state of U2585, which in turn precludes accommodation of the Lys-tRNA in the A-site and thus prevents peptide bond formation ( Fig. 5d ). In conclusion, our analysis of the ErmBL-SRC establishes a basic framework for understanding how the combined action of the nascent peptide and a small molecule cofactor may induce programmed translation arrest. It will be interesting to extend these insights by comparing the ErmBL-SRC structure with other drug-dependent SRCs, such as ErmCL, which have principally different antibiotic- and tunnel sensor requirements. Collectively, it appears that there are several alternative ways to inhibit translation via the cooperative action of nascent peptides and tunnel-binding antibiotics. Generation and purification of ErmBL-SRC The 2 × ermBL construct was synthesized (Eurofins, Martinsried, Germany) such that it contained a T7 promoter followed by a strong RBS spaced by 7 nucleotides (nts) to the ATG start codon of the first ermBL cistron ( Fig. 1a ). A linker of 22 nts separated the stop codon of the first ermBL cistron and the start codon of the second ermBL cistron ( Fig. 1c ). The linker also comprised the strong RBS 7 nts upstream of the ATG start codon of the second ermBL cistron, enabling initiation of translation independent from the first ermBL cistron ( Fig. 1c ). Each ermBL cistron encoded amino acids 1–17 corresponding to ErmBL leader peptide (Genbank accession number K00551) present on macrolide resistance plasmid pAM77 (ref. 29) [29] . The complete sequence of 2 × ermBL construct is: (T7 promoter, italics; RBS, bold; ErmBL ORF, shaded grey with GAT codon in P-site of stalled ribosome shown in bold; annealing site for complementary DNA oligonucleotide, underlined). In vitro translation of the 2 × ermBL construct was performed using the Rapid Translation System RTS 100 E. coli HY Kit (Roche; Cat. No. 3246817). Translations were carried out in the presence of 10 μM ERY for 1 h at 30 °C. Control reactions were performed in the absence of ERY as well as using a monocistronic ermBL construct ( Supplementary Fig. 1 ). Translation reactions were analysed on sucrose density gradients (10–55% sucrose in a buffer A, containing 50 mM HEPES-KOH, pH 7.4, 100 mM KOAc, 25 mM Mg(OAc) 2 , 6 mM β-mercaptoethanol, 10 μM ERY and 1 × Complete EDTA-free Protease Inhibitor cocktail (Roche)) by centrifugation at 154,693 g (SW-40 Ti, Beckman Coulter) for 2.5 h at 4 °C ( Fig. 1d ). For ErmBL-SRC purification, disome fractions were collected using a Gradient Station (Biocomp) with an Econo UV Monitor (Biorad) and a FC203B Fraction Collector (Gilson). Purified ErmBL-SRC disomes were concentrated by centrifugation using Amicon Ultra-0.5 ml Centrifugal Filters (Millipore) according to the manufacturer’s protocol. To obtain monosomes of the ErmBL-SRC, a short DNA oligonucleotide (5′-ttcctccttaaaact-3′, Metabion) was annealed to the linker between the ermBL cistrons of the disomes, generating a DNA–RNA hybrid that could be cleaved by RNase H (New England Biolabs) treatment in buffer A at 25 °C for 1 h ( Fig. 1c ). The RNase H-cleaved disome material was directly applied to the cryo-grids without any further purification. Aminoacylation status of tRNA Lys in the ErmBL-SRC RNA from three A 260 units of the disome peak, subjected to exactly the same procedures as required for preparation for cryo-EM, was extracted by acidic phenol, ethanol precipitated and dissolved in 6 μl NaOAc, pH 4.0. The isolated RNA was then resolved by electrophoresis in an 8 cm long (1 mm thick) 14% acidic denaturing gel [30] alongside with deacylated tRNA Lys and aminoacyl-tRNA markers. After electrophoresis for 24 h at 50 V in the cold room, the RNA was transferred to a Hybond N+ membrane (GE Healthcare) by electroblotting and probed with a [ 32 P]-5′-labelled DNA oligonucleotide complementary to tRNA Lys : (GTCGTGCAGGATTCGAACCTGCGACCAATTGATTAAAAGTCAACTGCTCTACCAACTGAGCTAACGACCC). Negative-stain EM Ribosomal particles were diluted in buffer A to a final concentration of 0.5 A 260 ml −1 . One drop of each sample was deposited on a carbon-coated grid. After 30 s, grids were washed with distilled water and then stained with three drops of 2% aqueous uranyl acetate for 15 s. The remaining liquid was removed by touching the grid with filter paper. Micrographs were taken using a Morgagni transmission electron microscope (FEI Company), 80 kV, wide angle 1 K charge-coupled device at direct magnifications of 72 K. Cryo-EM and single-particle reconstruction Monosomes of the ErmBL-SRC were applied to 2 nm pre-coated Quantifoil R3/3 holey carbon-supported grids and vitrified using a Vitrobot Mark IV (FEI Company). Data collection was performed on a Titan Krios transmission electron microscope (FEI Company) under low-dose conditions (about 20 e − per Å 2 ) at a nominal magnification of × 75,000 with a nominal defocus between −1 and −3.5 μm. Images were collected at 200 keV at a magnification of × 148,721 at the plane of charge-coupled device using a TemCam-F416 CMOS camera (TVIPS GmbH, 4,096 × 4,096 pixel, 15.6 μm pixel, 1 s per full frame), resulting in an image pixel size of 1.0605 Å (object scale). Data collection was facilitated by the semi-automated software EM-TOOLS (TVIPS GmbH) as described [31] . Contrast-transfer functions were determined using the SPIDER TF ED command and recorded images were manually inspected for good areas and power-spectra quality. Data were processed further using the SPIDER software package [32] , in combination with an automated workflow as described previously [31] . After initial, automated particle selection based on the programme SIGNATURE [33] , initial alignment was performed with 1,344,100 particles, using E. coli 70S ribosome as a reference structure [34] . After removal of noisy particles (527,625 particles; 39%), the data set could be sorted into three main subpopulations ( Supplementary Fig. 2 ) using an incremental K-means-like method of unsupervised 3D sorting [35] : the first subpopulation (353,318 particles; 26%) was defined by the presence of the L1 stalk adopting an ‘in’ conformation and the presence of non-stoichiometric density for tRNAs in the A-, P- and E-sites. The second and third subpopulations were defined by the presence of the L1 stalk adopting an ‘out’ conformation and the absence of density for the E-tRNA. The minor subpopulation contained only P-tRNA, but due to the small particle numbers (113,413 particles; 8%) could only be refined to ~7 Å resolution (with a Fourier shell correlation (FSC) cutoff of 0.5). In contrast, the major subpopulation (349,744 particles; 26%) contained both A- and P-tRNAs and could be refined to an average resolution of 6.6 Å (0.5 FSC) and a local resolution extending to 4.5 Å for the core of the 30S and 50S subunit ( Supplementary Fig. 3 ). Local resolution was computed within a softened sphere (radius of 22 Å) at each voxel, as described previously [36] , using the 0.5 FSC of two reconstructions; namely, from the first 50% of the particles and then the remaining 50%. Molecular modelling and map-docking procedures The molecular model for the ribosomal proteins and rRNA of the ErmBL-SRC was based on the 50S subunit from the crystal structure of ERY bound to the E. coli 70S ribosome (PDB3OFR) [11] and obtained by performing a rigid-body fit into the cryo-EM density map of the ErmBL-SRC using UCSF Chimera [37] (fit in map function). The conformations of 23S rRNA nucleotides U2584 and U2585 were taken from the equivalent nucleotides of the Haloarcula marismortui 50S subunit in complex with the unaccommodated A-site tRNA mimic (PDB1VQ6) [21] , [22] after the PDB was fitted as a rigid body into the ErmBL-SRC density map. The conformation of U2506 was similar to the equivalent nucleotide of the H. marismortui 50S subunit in complex with the accommodated A-site tRNA mimic (PDB1VQN) [21] , [22] , however, required manual rotation of the base to prevent clashing with the unaccommodated position of U2585. In contrast, the conformation of A2062 present in the ErmBL-SRC is unique, being distinct from the tunnel ‘in’ (PDB3CC2) [38] and tunnel ‘out’ (PDB1VQ6) [21] , [22] conformations observed in previously reported ribosome structures. The conformation of A2062 in the ErmBL-SRC is most closely related to conformations of this nucleotide observed in the Thermus thermophilus 70S ribosome (PDB2J01) [39] . To investigate the conformational state of the PTC of the ErmBL-SRC, crystal structures of H. marismortui 50S subunit in complex with model peptide bond substrates ( Fig. 5a,b ) were fitted into the cryo-EM density map of the ErmBL-SRC as a rigid body using UCSF Chimera [37] . The model for the ErmBL nascent polypeptide chain was generated and manually fitted into the density using Coot [40] . PDBs for the unaccommodated (PDB1VQ6) and accommodated (PDB1VQN) state of the PTC were filtered to 4.5 Å to using the Molmap function in Chimera. Difference electron density maps were then calculated by subtracting the filtered maps for 1VQ6 from 1VQN ( Supplementary Fig. 5a ) or ErmBL from 1VQN ( Supplementary Fig. 5b ). Figure preparation Figures showing electron densities and atomic models were generated using UCSF Chimera [37] . Toe-printing assay The DNA templates containing T7 promoter, RBS and the ErmBL-coding ORF (wild type or the mutants) were generated by crossover PCR. The toe-printing analysis of drug-dependent ribosome stalling was carried out as described [18] . Briefly, the DNA templates (0.1 pmol) were used in a total volume of 5 μl of PURExpress (New England Biolabs) cell-free transcription–translation reactions. Samples were incubated for 15 min at 37 °C, followed by addition of the [ 32 P]-labelled NV1 toe-printing primer designed to anneal ~100 nucleotides downstream from the anticipated ribosome-stalling site. The primer was extended by reverse transcriptase and the reaction products were analysed in sequencing gels. In experiments with mutant ribosomes, the ‘Δ ribosome’ version of the PUREXpress kit was supplemented with ribosomes (10 pmol per reaction) isolated from the SQ171 E. coli strain carrying the plasmid expressing E. coli rrnB operon with the engineered mutations in the 23S rRNA gene. Mutant ribosomes were purified as described [41] . Cell-free translation and analysis of peptidyl tRNA Translation of the ermBL ORF for peptidyl tRNA analysis was carried out in the E. coli S30 cell-free transcription–translation system (Promega). PCR-generated DNA template carrying the ermBL gene (shown in blue) under the control of the P tac promoter (green) had the following structure: The DNA template (0.1–0.5 pmol) was translated in a 5 μl reaction containing 100 μCi of [ 14 C]-Asp or [ 14 C]-Lys (specific activity of both: 208 mCi mmol −1 ) (American Radio Chemicals) following the manufacturer’s protocol. When required, translation reactions were carried out in the presence of 50 μM ERY or borrelidin. After 30 min incubation at 37 °C, samples were analysed in a 16% bis-tris polyacrylamide gel using MES running buffer (as described in http://openwetware.org/Sauer:bis-Tris_SDS_PAGE based on US patent 6,162,338). Gels were dried and exposed overnight to a phosphorimager screen. Accession codes : The cryo-EM map and associated molecular model of the ErmBL-SRC have been deposited in the EM databank under accession code EMD-5771 and the protein databank under PDB code 3J5L How to cite this article: Arenz, S. et al. Molecular basis for erythromycin-dependent ribosome stalling during translation of the ErmBL leader peptide. Nat. Commun. 5:3501 doi: 10.1038/ncomms4501 (2014).